Planar Möbius aromatic pentalenes incorporating 16 and 18 valence electron osmiums Aromaticity, a highly stabilizing feature of molecules with delocalized electrons in closed circuits, is generally restricted to ‘Hückel’ systems with 4 n +2 mobile electrons. Although the Möbius concept extends the principle of aromaticity to 4 n mobile electron species, the rare known examples have complex, twisted topologies whose extension is unlikely. Here we report the realization of osmapentalenes, the first planar Möbius aromatic complexes with 16 and 18 valence electron transition metals. The Möbius aromaticity of these osmapentalenes, documented by X-ray structural, magnetic and theoretical analyses, demonstrates the basis of the aromaticity of the parent osmapentalynes. All these osmapentalenes are formed by both electrophilic and nucleophilic reactions of the in-plane π component of the same carbyne carbon, illustrating ambiphilic carbyne reactivity, which is seldom observed in transition metal chemistry. Our results widen the scope of Möbius aromaticity dramatically and open prospects for the generalization of planar Möbius aromatic chemistry. Aromaticity, one of the most important concepts in chemistry, denotes the ‘extra’ stabilization of molecules because of electron delocalization in closed circuits [1] , [2] , [3] . Although Hückel aromatic compounds with 4 n +2 mobile electrons are common, examples of Möbius 4 n electrons aromaticity have proven to be much more difficult to realize and to establish [4] , [5] , [6] , [7] , [8] , [9] , [10] , [11] , [12] , [13] . Indeed, the reported Möbius aromatic compounds are very limited and almost all have twisted topologies [14] , [15] , [16] , [17] , [18] . For instance, although Heilbronner pointed out in 1964 that rings with 20 atoms or more might adopt Möbius geometries ‘without any apparent angle or steric repulsion strain’ in his prediction [4] , Mauksch et al. in 1998 discovered computationally a twisted much smaller ring system, the cyclononatetraenyl cation, which is a Möbius aromatic annulene [5] . Then Ajami et al. reported the first synthesis of a Möbius aromatic hydrocarbon in 2003, which also has a twisted topology [6] . Very recently, we reported osmapentalyne complexes [19] , persistent and highly unusual bicyclic systems via the strategy of the stabilization caused by a transition metal fragment [20] , [21] , [22] , [23] , [24] , [25] . This metal fragment not only relieves considerable ring strain in pentalyne, but also results in Möbius aromatic stabilization of the rarely realized planar Craig type, which was first proposed by Craig by analysing the interactions of d -atomic orbitals (AOs) present in an alternating cyclic array of main group p π- d π AOs by reference to trimeric and tetrameric phosphonitric chlorides [26] and was later extended to transition metal-containing 4 n π metallacycles by Mauksch and Tsogoeva computationally [27] . Interestingly, the metal–carbon triple bond in osmapentalynes can shift from one five-membered ring to another [19] . We speculated that a protonation–deprotonation process via an osmapentalene intermediate could account for this tautomerization ( Fig. 1a ). Because the in-plane π-electrons of the triple bonds do not contribute to the aromaticity of osmapentalynes, Möbius aromaticity in osmapentalynes should be rooted in osmapentalenes. Therefore, osmapentalenes were also expected to exhibit Möbius aromaticity. 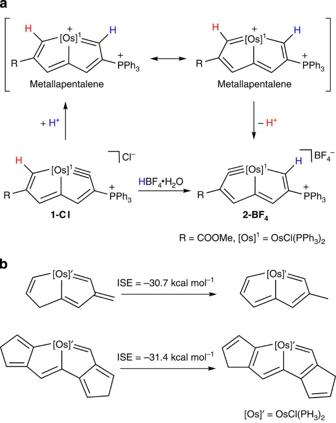Figure 1: The proposed aromatic metallapentalene. (a) The 16-electron osmapentalene intermediate proposed in the tautomeric metal–carbon triple bond shift of osmapentalyne. (b) The aromaticity of a model osmapentalene evaluated by the two variations of the ISE method. The energies (computed by the B3LYP functional with the LanL2DZ basis set for osmium and the 6-311++G(d,p) basis sets for carbon and hydrogen) include zero-point energy corrections. ISE, isomerization stabilization energy. Figure 1: The proposed aromatic metallapentalene. ( a ) The 16-electron osmapentalene intermediate proposed in the tautomeric metal–carbon triple bond shift of osmapentalyne. ( b ) The aromaticity of a model osmapentalene evaluated by the two variations of the ISE method. The energies (computed by the B3LYP functional with the LanL2DZ basis set for osmium and the 6-311++G(d,p) basis sets for carbon and hydrogen) include zero-point energy corrections. ISE, isomerization stabilization energy. Full size image Although six-coordinated transition metal complexes with octahedral structures are expected to follow the 18-electron transition metal rule [28] , protonation of the carbyne carbon of osmapentalyne results in an aromatic osmapentalene having an osmium with only 16 electrons. Could the magnitude of the Möbius aromaticity be sufficient to overwhelm the instability associated with this 18-electron rule violation? Herein, we report the actual isolation of the first 16-electron metallapentalene, a rare Möbius aromatic system with a planar, rather than a twisted topology. Synthesis of the first 16-electron metallapentalene We first evaluated the ‘isomerization stabilization energy’ (ISE) using effective variations of the Schleyer–Pühlhofer method [29] , [30] . The ISE values of osmapentalene in Fig. 1b , −30.7 and −31.4 kcal mol −1 , are very close to the corresponding ISE values of benzene (−33.2 and −29.0 kcal mol −1 ) [29] , [30] and even larger than those of osmapentalyne (−21.2 and −19.6 kcal mol −1 ) [19] . Therefore, we reasoned that it might be possible to detect or even to trap the intermediate, 16-electron osmapentalene. Indeed, treating either 1-Cl or 2-BF 4 with HBF 4 ·Et 2 O at room temperature for 30 min led in both cases to 16-electron osmapentalene 3-(BF 4 ) 2 ( Fig. 2a ), which was isolated quantitatively as a yellow solid. However, as a 16-electron osmium complex, 3-(BF 4 ) 2 is prone to conversion into osmapentalynes with an 18-electron osmium centre. When 3-(BF 4 ) 2 was treated with Et 2 O, osmapentalynes 1-BF 4 and 2-BF 4 were formed in a 7:93 ratio based on the 1 H nuclear magnetic resonance (NMR) spectroscopy. Density functional theory computations were employed to investigate the mechanism for the formation of osmapentalynes 1-BF 4 and 2-BF 4 from osmapentalene 3-(BF 4 ) 2 . The PPh 3 s were replaced by PH 3 s. As shown in Fig. 3 , deprotonation of osmapentalene 3′ at the C1 and C7 carbon atoms only have 12.1 and 7.0 kcal mol −1 free energy reaction barriers, respectively, leading to the formation of osmapentalynes 1′ and 2′ . Our results also indicate that osmapentalyne 2′ is thermodynamically more stable than osmapentalyne 1′ in line with the experimental observations that osmapentalyne 2-BF 4 was the major product. 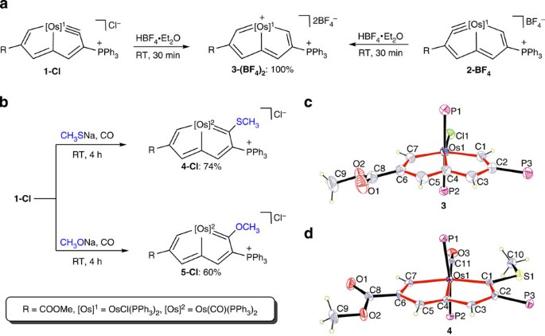Figure 2: Synthesis of 16- and 18-electron osmapentalenes. (a) The protonation of osmapentalyne gives 16-electron osmapentalene3-(BF4)2. (b) Reactions of osmapentalyne1-Clwith nucleophiles, leading to the formation of 18-electron osmapentalenes4-Cland5-Cl. (c,d) X-ray structures of3(c) and4(d) (drawn with 50% probability). Phenyl moieties in PPh3have been omitted for clarity. Selected bond lengths (Å) for3: Os1–C1 1.978(6), Os1–C4 2.139(6), Os1–C7 1.926(6), C1–C2 1.365(9), C2–C3 1.414(9), C3–C4 1.376(9), C4–C5 1.404(9), C5–C6 1.378(9), C6–C7 1.393(9). Selected bond lengths (Å) for4: Os1–C1 2.080(4), Os1–C4 2.083(3), Os1–C7 2.081(4), Os1–C11 1.914(4), C1–C2 1.457(5), C2–C3 1.399(5), C3–C4 1.389(5), C4–C5 1.378(5), C5–C6 1.407(5), C6–C7 1.377(5), C1–S1 1.733(4), S1–C10 1.787(4), C11–O3 1.141(4). RT, room temperature. Figure 2: Synthesis of 16- and 18-electron osmapentalenes. ( a ) The protonation of osmapentalyne gives 16-electron osmapentalene 3-(BF 4 ) 2 . ( b ) Reactions of osmapentalyne 1-Cl with nucleophiles, leading to the formation of 18-electron osmapentalenes 4-Cl and 5-Cl . ( c , d ) X-ray structures of 3 ( c ) and 4 ( d ) (drawn with 50% probability). Phenyl moieties in PPh 3 have been omitted for clarity. Selected bond lengths (Å) for 3 : Os1–C1 1.978(6), Os1–C4 2.139(6), Os1–C7 1.926(6), C1–C2 1.365(9), C2–C3 1.414(9), C3–C4 1.376(9), C4–C5 1.404(9), C5–C6 1.378(9), C6–C7 1.393(9). Selected bond lengths (Å) for 4 : Os1–C1 2.080(4), Os1–C4 2.083(3), Os1–C7 2.081(4), Os1–C11 1.914(4), C1–C2 1.457(5), C2–C3 1.399(5), C3–C4 1.389(5), C4–C5 1.378(5), C5–C6 1.407(5), C6–C7 1.377(5), C1–S1 1.733(4), S1–C10 1.787(4), C11–O3 1.141(4). RT, room temperature. 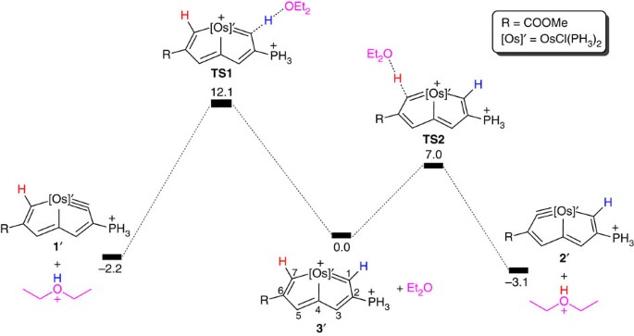Figure 3: Reaction mechanism for the formation of1′and2′from3′. The computed free energies are in kcal mol−1. Full size image Figure 3: Reaction mechanism for the formation of 1′ and 2′ from 3′ . The computed free energies are in kcal mol −1 . Full size image The structure of 3-(AlCl 4 ) 2 in the solid state (generated from the reaction of 1-Cl or 2-BF 4 with AlCl 3 in wet dichloromethane) has been verified by X-ray diffraction ( Supplementary Fig. 1 and Supplementary Data 1 ). As shown in Fig. 2c , the metallabicycle moiety of 3 is almost planar. The mean deviation from the least-squares plane is only 0.0106 Å. The Os1–C1 (1.978 Å) and Os1–C7 (1.926 Å) bond lengths are in the range of Os−C bond lengths (1.894−2.080 Å) of osmabenzene [31] , [32] . The Os1−C4 (2.139 Å) bond length is longer than other Os−C bond lengths, in line with the resonance structures depicted in Supplementary Fig. 2 , in which Os1−C4 is always a single σ-bond, similar to the previous observation in osmapentalynes [19] . Distances of C−C bonds (1.365–1.414 Å) of the fused five-membered rings are between C−C single- and double-bond lengths, indicating a delocalized structure [33] , [34] , [35] , [36] , [37] , [38] , [39] , [40] , [41] , [42] . Complex 3-(BF 4 ) 2 was further characterized by 1 H, 31 P and 13 C NMR spectroscopy. The low field H1 and H7 resonances at 12.08 and 11.94 parts per million (p.p.m. ), respectively, are particularly noteworthy. The H3 and H5 signals at 9.48 and 9.04 p.p.m., respectively, are also downfield. The 31 P NMR spectrum of 3-(BF 4 ) 2 displays a triplet signal at 11.97 p.p.m. for C P Ph 3 and a doublet signal at 29.15 p.p.m. for two equivalent Os P Ph 3 . The metal-bound C1, C4 and C7 signals are downfield, at 226.9, 194.6 and 244.2 p.p.m., respectively. The downfield 1 H chemical shifts, the delocalized metal–carbon and carbon–carbon bonds, and the near-perfect planarity of the fused five-membered rings, vindicate the aromaticity in 16-electron osmapentalene 3 . Additional confirmation of the aromatic nature of osmapentalene 3 was provided by canonical molecular orbital (CMO) nucleus-independent chemical shift (NICS) [43] , [44] , [45] computations [46] on the simplified unsubstituted model complex 3″ , where PH 3 s replace the PPh 3 ligands. The negative NICS(0) zz (−11.3 p.p.m.) values at the centres of each ring in 3″ approach the benzene value (−14.5 p.p.m.) and are in sharp contrast with those of pentalene (+91.2 p.p.m.). As shown in Fig. 4 , four of the five occupied π MOs of 3″ (HOMO, HOMO-2, HOMO-8 and HOMO-11) reflect the π delocalization along the perimetre of the bicyclic system. Specifically, three MOs (HOMO, HOMO-1 and HOMO-11) are derived from the orbital interactions between the p zπ AOs of the C 7 H 6 unit (perpendicular to the bicycle plane) and the 5 d xz orbital of the Os atom, whereas two MOs (HOMO-2 and HOMO-8) are formed by the orbital interactions between the p zπ AOs of the C 7 H 6 unit and the 5 d yz orbital of the Os atom. The overall Möbius aromaticity of the model complex 3″ can be attributed to the total diamagnetic contributions from the four orbitals (HOMO, HOMO-2, HOMO-8 and HOMO-11). Thus, this is the first extension of Möbius aromaticity to a planar 16-electron complex. The positive NICS(0) zz value of HOMO-1 (+4.5) is consistent with its lack of ‘perimetre character’. Despite its π character shown in HOMO-1, Os–C4 has the smallest Wiberg bond index among the three Os–C bonds in 3″ . Specifically, the Wiberg bond indices of Os–C1, Os–C4 and Os–C7 are 0.97, 0.57 and 0.97, respectively. The smallest Wiberg bond index of Os–C4 is in line with the experimental observation that Os–C4 in osmapentalene 3 has the longest metal–carbon bond distance ( Fig. 2c ). 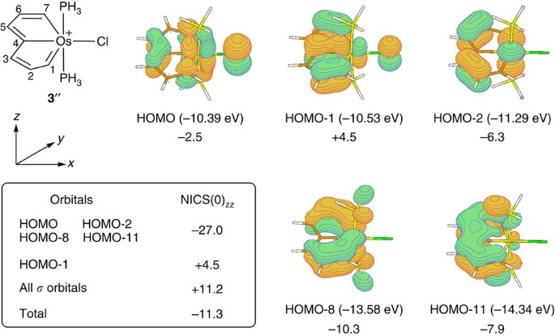Figure 4: NICS(0)zzcontributions of π molecular orbitals (MOs) of 3″(C2v). Note that HOMO-1 is not a perimetre MO and does not contribute to the aromaticity. The eigenvalues of the MOs are given in parentheses and the nucleus-independent chemical shift (NICS) values in p.p.m. Figure 4: NICS(0) zz contributions of π molecular orbitals (MOs) of 3 ″ (C 2v ). Note that HOMO-1 is not a perimetre MO and does not contribute to the aromaticity. The eigenvalues of the MOs are given in parentheses and the nucleus-independent chemical shift (NICS) values in p.p.m. Full size image Synthesis of 18-electron osmapentalenes As 16-electron osmapentalene 3-(BF 4 ) 2 has been achieved by protonation of complex 1 - Cl ( Fig. 2a ), 18-electron osmapentalenes might be accessible if nucleophiles can also attack the carbyne carbon of complex 1 - Cl . Indeed, the methanethiolate (CH 3 S – ) and the methanolate (CH 3 O – ) anions react with osmapentalyne 1 - Cl to generate osmapentalenes 4 - Cl and 5 - Cl under CO atmospheres at room temperature for 4 h ( Fig. 2b ). All these new osmapentalenes are remarkably persistent. Thus, no significant decomposition of a sample of 4 - Cl occurred even after heating in air at 170 °C for at least 5 h. For these two osmapentalenes, we also examined their ultraviolet–visible absorption spectra ( Supplementary Fig. 3 ). The maximum absorption of 4-Cl in the visible region was located at 505 nm, with a slight red shift by 40 nm relative to 5-Cl ( λ max =465 nm). Both of the maximum absorptions of osmapentalenes 4-Cl and 5-Cl in the visible region have a red shift in comparison with osmapentalyne [19] . The structure of osmapentalene 4 - Cl has also been characterized by NMR spectroscopy and high-resolution mass spectrometry (HRMS). The singlet 1 H NMR signal at 12.46 p.p.m. is assigned to the OsC H proton. The H3 and H5 signals were located at 8.36 and 8.01 p.p.m., respectively. The spectrum displayed the signals of the four metal-bound 13 C NMR carbon atoms at 242.8 (C1), 213.8 (C7), 195.5 (C4) and 191.0 (Os– C O) p.p.m. The 13 C NMR signal of S C H 3 was observed at 28.7 p.p.m. In the 31 P NMR spectrum of 4 - Cl , C P Ph 3 resonates at 10.07 p.p.m. as a triplet, and two equivalents Os P Ph 3 appear as a doublet at 3.54 p.p.m. Single-crystal X-ray diffraction established the solid-state structure of osmapentalene 4 - Cl . As shown in Fig. 2d (also in Supplementary Fig. 4 and Supplementary Data 2 ), its two fused five-membered rings are nearly coplanar; the mean deviation from the least-squares plane is only 0.0274 Å. The almost equal Os–C bond lengths in the two fused five-membered rings (2.080 Å, Os1–C1; 2.083 Å, Os1–C4 and 2.081 Å, Os1–C7) indicate a delocalized structure. The Os1–C11 (1.914 Å) bond length is within the typical Os–C double bond range (1.775–2.144 Å) [31] . The C11–O3 (1.141 Å) length is in the range of the M=C=O carbonyl bond lengths (1.148–1.272 Å) [31] . The structure of osmapentalene 5 - Cl was fully supported by NMR spectroscopy, HRMS and X-ray diffraction ( Supplementary Fig. 5 and Supplementary Data 3 ). The structural features and dimensions of the metallabicycle are very similar to those of 4 and contrast with the nonplanar rings of an analogous iridabicycle, metallabicyclooctatriene complex [47] . The delocalized Os–C and C–C bond lengths together with the planarity of the fused five-membered ring support the aromaticity of 18-electron osmapentalenes 4 - Cl and 5 - Cl . The ISE method also confirmed and evaluated the aromaticity of a simplified unsubstituted C 2v symmetry model complex 4″ (of the 18-electron osmapentalenes 4 - Cl and 5 - Cl in Fig. 2b ) where PH 3 s replace the PPh 3 ligands. The ISE reactions chosen in Fig. 5 have the same total number of anti -diene units in the reactants and in their products. The large negative energy of the first reaction (–25.7 kcal mol −1 ) is approximately four-fifths of benzene’s ISE (–33.2 kcal mol −1 ) value [29] , in sharp contrast to the positive (8.8 kcal mol −1 ) pentalene value [19] . The second reaction in Fig. 5 employing another strain-balanced isomerization method [30] , evaluates a –23.4 kcal mol −1 aromatic stabilization energy. This result for osmapentalene is also approximately four-fifths that of benzene (–29.0 kcal mol −1 ) using the same approach [30] . The two highly negative ISE values in Fig. 5 confirm the osmapentalene aromaticity unambiguously. 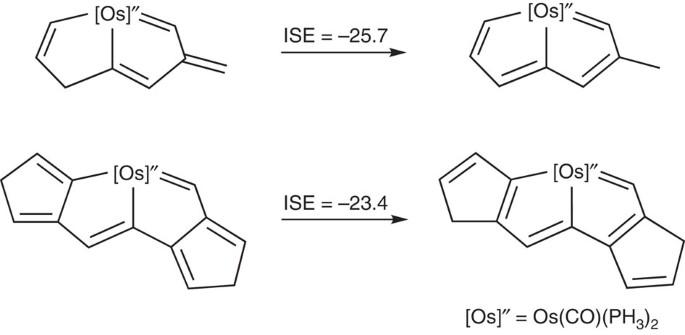Figure 5: Isomerization stabilization energy (ISE) evaluations of the aromaticity of4″. The aromaticity evaluated by the two variations of the ISE method. The energies (in kcal mol−1computed by the B3LYP functional with the LanL2DZ basis set for osmium and the 6-311++G(d,p) basis sets for carbon and hydrogen) include zero-point energy corrections. Figure 5: Isomerization stabilization energy (ISE) evaluations of the aromaticity of 4″ . The aromaticity evaluated by the two variations of the ISE method. The energies (in kcal mol −1 computed by the B3LYP functional with the LanL2DZ basis set for osmium and the 6-311++G(d,p) basis sets for carbon and hydrogen) include zero-point energy corrections. Full size image CMO-NICS computations on model complex 4″ agree. The −8.4 p.p.m. NICS(0) zz at the centre of each ring of 4″ ( Fig. 6 ), approaches the −11.3 p.p.m. value of osmapentalene 3″ and contrasts sharply with the +91.2 p.p.m. of pentalene. Notably, the Os–C11 Wiberg bond index (0.97) in 4″ is much larger than that of Os–C1 (0.65), Os–C4 (0.42) and Os–C7 (0.65). Therefore, Os–C11 has some double bond character; its experimental bond length is shortest among the four Os–C bonds. 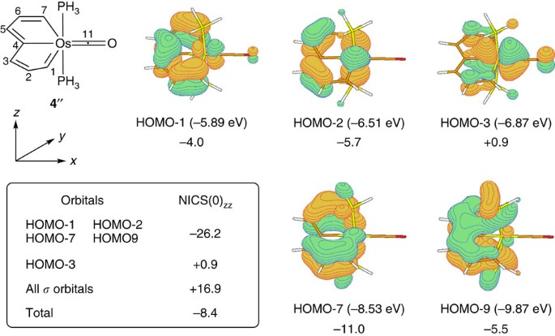Figure 6: NICS(0)zzcontributions of π molecular orbitals (MOs) of 4'' (C2v). Note that HOMO-3 is not a perimetre MO and does not contribute to the aromaticity. The eigenvalues of the MOs are given in parentheses and the nucleus-independent chemical shift (NICS) values in p.p.m. Figure 6: NICS(0) zz contributions of π molecular orbitals (MOs) of 4'' (C 2v ). Note that HOMO-3 is not a perimetre MO and does not contribute to the aromaticity. The eigenvalues of the MOs are given in parentheses and the nucleus-independent chemical shift (NICS) values in p.p.m. Full size image Like 3″ ( Fig. 4 ), the five occupied π MOs of 4″ in Fig. 6 can be derived principally from the orbital interactions between the p zπ AOs of the C 7 H 6 unit and two of the d orbitals of the Os atom (5 d xz and 5 d yz ). Three of the MOs shown in Fig. 6 (HOMO-1, HOMO-3 and HOMO-9) are derived from the orbital interactions between the p zπ AOs of the C 7 H 6 unit and the 5 d xz orbital of the Os atom, whereas two MOs (HOMO-2 and HOMO-7) are formed by the orbital interactions between the p zπ AOs of the C 7 H 6 unit and the 5 d yz (Os) orbital. Again, the Möbius aromaticity of the model complex 4″ can be attributed to the total diamagnetic contributions (−26.2 p.p.m.) from the four MOs (HOMO-1, HOMO-2, HOMO-7 and HOMO-9; Fig. 6 ). Note that a ‘localized’ d xz orbital is located in HOMO-3 compared with other MOs, leading to a positive NICS(0) zz value (+0.9). We isolated the reaction intermediate, osmapentalene, involved in the shift of the Os≡C triple bond between osmapentalynes rings. This first-known aromatic metallapentalene was synthesized by the addition of electrophile to osmapentalyne even though its osmium only has 16 valence electrons. Osmapentalenes with 18 valence electrons osmiums were also prepared by the addition of nucleophiles to osmapentalynes, thus demonstrating the amphiphilic reactivity of the same carbyne carbon, which is seldom observed in organometallic chemistry. Theoretical computations reveal that all these osmapentalenes with planar metallacycle benefit from Craig–Möbius aromaticity, which appears to be more important than the 16 or 18 valence electrons count. Our achievement reveals that the Möbius aromaticity in osmapentalynes is rooted in osmapentalenes. As Craig–Möbius aromaticity [26] , [27] was first proposed in 1958, authentic examples of planar Möbius aromaticity are very rare. The realization of osmapentalynes [19] and osmapentalenes has widened the scope of Möbius aromaticity significantly and opens a new avenue for the construction of other planar Möbius aromatic complexes. General considerations All syntheses were carried out under an inert atmosphere (N 2 ) by means of standard Schlenk techniques. Solvents were distilled from sodium/benzophenone (hexane) or calcium hydride (dichloromethane and 1,2-dichloroethane) under N 2 before use, unless otherwise stated. The metallapentalyne was synthesized according to the previously published procedure [19] . Other reagents were used as received from commercial sources without further purification. Further experimental details and the synthesis procedures for 3-(AlCl 4 ) 2 and 5-Cl are described in the Supplementary Methods . The procedures for 3-(BF 4 ) 2 and 4-Cl are described below. Two-dimensional and one-dimensional NMR are abbreviated as heteronuclear single quantum coherence (HSQC), heteronuclear multiple bond correlation (HMBC), and distortionless enhancement by polarization transfer (DEPT). All of the NMR spectra can be found in the Supplementary Figs 6–20 . Synthesis of osmapentalene 3-(BF 4 ) 2 A solution of HBF 4 ·Et 2 O (53 μl, 0.20 mmol) was added to a solution of 1-Cl (203 mg, 0.17 mmol) or 2-BF 4 (212 mg, 0.17 mmol) in dichloromethane (10 ml). After stirring at room temperature for 30 min, the mixture was dried under vacuum to give 3-(BF 4 ) 2 (226 mg, 100%) as a yellow solid. 1 H-NMR plus 1 H– 13 C HSQC (500 MHz, CD 2 Cl 2 ): δ =12.08 (s, 1H, H1), 11.94 (s, 1H, H7), 9.48 (s, 1H, H3), 9.04 (s, 1H, H5), 3.99 (s, 3H, COOC H 3 ), 8.25–7.17 p.p.m. (m, 45H, PPh 3 ). 31 P-NMR (202 MHz, CD 2 Cl 2 ): δ =29.15 p.p.m. (d, J P-P =4.9 Hz, Os P Ph 3 ), 11.97 (t, J P-P =4.9 Hz, C P Ph 3 ). 13 C-NMR plus DEPT-135 and 1 H– 13 C HSQC (126 MHz, CD 2 Cl 2 ): δ =244.2 (br, C7), 226.9 (br, C1), 194.6 (d, J P-C =17.8 Hz, C4), 163.1 (s, C5), 160.5 (s, C OOCH 3 , confirmed by 1 H– 13 C HMBC), 158.6 (d, J P-C =13.3 Hz, C3), 157.4 (s, C6), 115.5 (d, J P-C =91.3 Hz, C2), 63.9 (s, COO C H 3 ), 141.3–125.3 p.p.m. (m, PPh 3 ). Analysis (calcd, found for C 63 H 52 ClB 2 F 8 O 2 OsP 3 ): C (56.75, 56.81), H (3.93, 4.02). Synthesis of osmapentalene 4-Cl A mixture of 1-Cl (203 mg, 0.17 mmol) and CH 3 SNa (35 mg, 0.50 mmol) in dichloromethane (10 ml) was stirred under CO atmosphere at room temperature for 4 h to give a red solution and then the solid suspension was removed through a filtre. The filtrate was concentrated to ca 2 ml and then purified by column chromatography (neutral alumina, eluent: dichloromethane/methanol=20:1) to give a red solution. The red solid of 4-Cl (155 mg, 74%) was collected after the solvent was evaporated to dryness under vacuum. 1 H-NMR plus 1 H– 13 C HSQC (400 MHz, CDCl 3 ): δ =12.46 (s, 1H, H7), 8.36 (d, J P-H =6.8 Hz, 1H, H3), 8.01 (s, 1H, H5), 3.53 (s, 3H, COOC H 3 ), 2.10 (s, 3H, SC H 3 ), 7.84–7.05 p.p.m. (m, 45H, PPh 3 ). 31 P-NMR (162 MHz, CDCl 3 ): δ =10.07 (t, J P-P =4.0 Hz, C P Ph 3 ), 3.54 p.p.m. (d, J P-P =4.0 Hz, Os P Ph 3 ). 13 C-NMR plus DEPT-135 and 1 H– 13 C HSQC (101 MHz, CDCl 3 ): δ =242.8 (br, C1), 213.8 (t, J P-C =13.1 Hz, C7), 195.5 (dt, J P-C =25.5 Hz, J P-C =6.1 Hz, C4), 191.0 (t, J P-C =11.1 Hz, Os C O), 168.2 (d, J P-C =21.0 Hz, C3), 163.9 (s, C OOCH 3 , confirmed by 1 H– 13 C HMBC), 160.0 (s, C5), 159.1 (s, C6), 120.9 (d, J P-C =86.5 Hz, C2), 51.5 (s, COO C H 3 ), 28.7 (s, S C H 3 ), 135.0–128.0 p.p.m. (m, PPh 3 ). Analysis (calcd, found for C 65 H 54 ClSO 3 OsP 3 ): C (63.28, 63.61), H (4.41, 4.74). HRMS (electrospray ionization (ESI)): m/z calcd for [C 65 H 54 O 3 OsP 3 S] + , 1199.2621; found, 1199.2624. X-ray crystallographic analysis Single crystals suitable for X-ray diffraction were grown from dichloromethane ( 3-(AlCl 4 ) 2 and 5-Cl ) or dichloroethane ( 4-Cl ) solution layered with hexane. Diffraction data were collected on a Rigaku R-AXIS SPIDER IP charge-coupled device (CCD) area detector ( 3-(AlCl 4 ) 2 and 5-Cl ) or on an Oxford Gemini S Ultra CCD area detector ( 4-Cl ) using graphite-monochromated Mo Kα radiation ( λ =0.71073 Å). Semi-empirical or multi-scan absorption corrections (SADABS) were applied [48] . All structures were solved by the Patterson function, completed by subsequent difference Fourier map calculations and refined by full matrix least-squares on F 2 with all the data using the SHELXTL programme package [49] . All non-hydrogen atoms were refined anisotropically unless otherwise stated. Hydrogen atoms were placed at idealized positions and assumed the riding model. See Supplementary Methods for the crystal data details of complexes 3-(AlCl 4 ) 2 , 4-Cl and 5-Cl. Computational details All structures were optimized at the B3LYP level of density functional theory [50] , [51] , [52] . In addition, the frequency calculations were performed to confirm the characteristics of the calculated structures as minima or transition states. In the B3LYP calculations, the effective core potentials of Hay and Wadt with a double-ζ valence basis set (LanL2DZ) were used to describe the Os, P and Cl atoms, whereas the standard 6–311++G(d,p) basis set was used for the C and H atoms [53] for all the ISE calculations. For these calculations described in Fig. 3 , we used the 6–31G(d) basis set for C, O and H atoms and optimized all the structures using the PCM model with dichloromethane as the solvent [54] , [55] , [56] , [57] . Polarization functions were added for Os ( ζ ( f )=0.886), Cl ( ζ ( d )=0.514) and P ( ζ ( d )=0.34) [58] in all the calculations. NICS values were calculated at the B3LYP-GIAO/6-311++G(d,p) level. All the optimizations were performed with the Gaussian 03 software package [59] , whereas the CMO-NICS calculations were carried out with the NBO 5.0 programme [46] interfaced with the Gaussian 98 programme [60] . See the Supplementary Data 4 for the Cartesian coordinates. Accession codes: The X-ray crystal structure information is available at the Cambridge Crystallographic Data Centre (CCDC) under deposition numbers CCDC-845145 ( 3-(AlCl 4 ) 2 ), CCDC-954860 ( 4-Cl ) and CCDC-954861 ( 5-Cl ). These data can be obtained free of charge from The Cambridge Crystallographic Data Centre via http:// www.ccdc.cam.ac.uk/data_request/cif . How to cite this article: Zhu, C. et al. Planar Möbius aromatic pentalenes incorporating 16 and 18 valence electron osmiums. Nat. Commun. 5:3265 doi: 10.1038/ncomms4265 (2014).